Transparent and flexible low noise graphene electrodes for simultaneous electrophysiology and neuroimaging Calcium imaging is a versatile experimental approach capable of resolving single neurons with single-cell spatial resolution in the brain. Electrophysiological recordings provide high temporal, but limited spatial resolution, because of the geometrical inaccessibility of the brain. An approach that integrates the advantages of both techniques could provide new insights into functions of neural circuits. Here, we report a transparent, flexible neural electrode technology based on graphene, which enables simultaneous optical imaging and electrophysiological recording. We demonstrate that hippocampal slices can be imaged through transparent graphene electrodes by both confocal and two-photon microscopy without causing any light-induced artefacts in the electrical recordings. Graphene electrodes record high-frequency bursting activity and slow synaptic potentials that are hard to resolve by multicellular calcium imaging. This transparent electrode technology may pave the way for high spatio-temporal resolution electro-optic mapping of the dynamic neuronal activity. Studying the complex wiring of neural circuits within human brain is critical for understanding cognitive functions, and is also vital in developing targeted treatments for neurological and psychiatric disorders. In the past two decades, breakthroughs in neuro-imaging have leveraged our understanding by generating high-resolution wiring diagrams of the brain [1] , [2] , [3] , [4] . Functional optical imaging of brain tissue has been shown to provide tremendous information on the dynamic properties of multiple cells (>100) simultaneously [5] , [6] . However, fully decoding the functions of individual circuit elements requires simultaneous information on the identity, spatial location and wiring of neurons, as well as their firing patterns, with great precision. Simultaneous electrophysiology and optical imaging could leverage the temporal and spatial resolution advantages of both techniques. Metal microelectrode arrays commonly used for recording neural activity cannot be used for such purposes, as they block the field of view, generate optical shadows and are prone to producing light-induced artefacts in the recordings. Completely transparent microelectrodes can offer a solution for this spatial-temporal resolution dilemma by enabling simultaneous imaging and electrophysiology from the same microcircuit. In addition, scaling down microelectrode dimensions while maintaining a high enough signal-to-noise ratio (SNR) to faithfully transduce cellular activity has been a major challenge. There have been several promising attempts to build transparent electrodes using indium tin oxide [7] , [8] , [9] . Indium tin oxide is a very expensive and brittle material, which cracks easily upon bending, making it unsuitable for flexible electrode arrays. Partially transparent transistors [10] have also been fabricated, however, their opaque source, drain and interconnects make them unsuitable for imaging larger areas or neural circuits [10] . Although microscopy techniques used for calcium imaging have generally a small field of view, complete transparency over larger areas is critical to use them with wide-field voltage imaging or in serial calcium imaging experiments to correlate small-scale and large-scale dynamic networks. As of yet, neural recordings with completely transparent, flexible electrode arrays, compatible with in vitro and in vivo imaging techniques, have not been demonstrated, to our knowledge. Novel material systems, such as emerging two-dimensional materials, carbon nanotube composites [11] , nanowires [12] and PEDOT:PSS [13] , which may provide flexibility and transparency for simultaneous optical imaging and electrophysiology, need to be explored. We investigated graphene, an emerging two-dimensional material, to build low noise, transparent and flexible neural electrodes. Graphene has recently emerged as the most investigated two-dimensional material, owing to its unique band structure and superior electrical [14] , mechanical [15] and thermal properties [16] . Successful growth of large-area graphene has facilitated efforts to use it as a transparent electrode material in flexible displays [17] , [18] and solar cells [19] . Mechanical characteristics [15] and flexibility of graphene have been extensively investigated for numerous applications including flexible batteries [20] , super capacitors [21] , sensors [22] , displays and flexible electronics [23] , [24] . Graphene devices also have low electronic noise, leading to sensor technologies with unprecedented sensitivities, enabling detection of individual molecules [25] , [26] . Promising results for graphene biocompatibility increase its potential use in biomedical applications [27] , [28] , [29] , [30] as well. Different from other transparent conducting materials, graphene uniquely combines flexibility, low noise and protection against corrosion [31] , [32] in one single-material system. Flexibility is particularly important for compatibility with advanced in vivo microscopy techniques in freely behaving animals [33] . Here we describe a neural electrode technology based on graphene for simultaneous optical imaging and electrophysiological recording. We have developed micro-fabrication techniques to build transparent graphene microelectrodes on flexible substrates. Electrical characterizations and in vivo neural recording experiments show that graphene electrodes can achieve a significant improvement in SNR and substantial reduction in electrical interference noise compared with gold electrodes. We demonstrate that transparent graphene electrodes can simultaneously record neural activity during calcium imaging with confocal or multiphoton microscopy without any laser-induced artefacts in the recordings. Combination of both techniques reveals temporal and spatial characteristics of high-frequency bursting activity and synaptic potentials in hippocampal slices with high precision. Fabrication and characterization of graphene electrodes Motivated by the flexibility, transparency and low noise characteristics of graphene, we fabricated graphene microelectrodes on flexible polyimide (Kapton) substrates ( Fig. 1a ). Graphene grown on copper (Cu) by chemical vapour deposition was transferred onto polyimide substrate with previously patterned gold (Au) contacts. Following the patterning of graphene, SU-8 was deposited as an encapsulation layer, covering the whole surface except electrode sites. As control samples, bare gold and non-transparent graphene/gold (G/Au) electrodes were fabricated along with the graphene using the same process flow. Graphene samples were doped with nitric acid. Details of the electrode fabrication are provided in the Methods and Supplementary Material ( Supplementary Fig. 1 ). Single electrodes were fabricated for electrochemical characterization ( Supplementary Fig. 2a,b ). Arrays were designed for in vivo electrocorticography recordings and in vitro hippocampal slice recordings ( Supplementary Fig. 2c,d ). 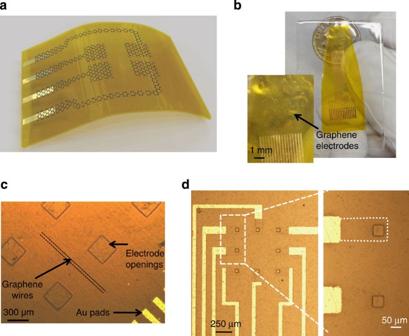Figure 1: Description of graphene electrodes. (a) Schematic illustration of a flexible graphene neural electrode array. Patterned graphene electrodes are in contact with Au contact pads to interface with the data acquisition system. (b) Photograph of a 16-electrode transparent array. The electrode size is 300 × 300 μm2. Inset, a closer view showing the electrode area. Fainted squares are the electrode openings in the encapsulation layer. (c) Microscope image of the array inb. Fainted patterns of graphene electrodes and wires are visible. (d) Microscope image of an 8-electrode hippocampal slice array. The electrode size is 50 × 50 μm2. Figure 1b,c shows images of a cortical electrocorticography array. Figure 1d shows a microscopic image of a hippocampal slice array with 50 × 50 μm 2 electrode area. Although graphene provides weak optical contrast, patterning graphene with oxygen plasma etching changes the surface characteristics of polyimide and results in faded patterns, which are slightly visible under optical microscope. In addition to surface electrodes, penetrating depth electrodes can also be designed and fabricated using the same fabrication processes. Thickness, material characteristics and geometry of the polyimide substrate can be engineered to provide enough stiffness to penetrate in brain tissue ( Supplementary Fig. 3a,b ). In an alternative approach, a thin flexible substrate bonded to a stiff carrier microneedle [34] can be utilized to implant the flexible electrode to desired depths. After penetrating to the desired depth, the microneedle will be separated from the flexible substrate and removed from the tissue. Figure 1: Description of graphene electrodes. ( a ) Schematic illustration of a flexible graphene neural electrode array. Patterned graphene electrodes are in contact with Au contact pads to interface with the data acquisition system. ( b ) Photograph of a 16-electrode transparent array. The electrode size is 300 × 300 μm 2 . Inset, a closer view showing the electrode area. Fainted squares are the electrode openings in the encapsulation layer. ( c ) Microscope image of the array in b . Fainted patterns of graphene electrodes and wires are visible. ( d ) Microscope image of an 8-electrode hippocampal slice array. The electrode size is 50 × 50 μm 2 . Full size image The low noise and high electrical conductivity of graphene can provide a promising route for scaling electrode size to single-cell dimensions by improving the SNR, reducing the electrical impedance and improving charge injection capacity. Furthermore, enhancing the out of plane conductivity of graphene is very important for electrochemical sensing applications. Chemical doping [35] , [36] , [37] techniques have been developed to reduce the sheet resistance of graphene. By exposing the graphene surface to nitric acid, adsorption of the electropositive NO 3 − groups on the graphene surface results in p-type doping. Electrochemical impedance spectroscopy (EIS) measurements performed on graphene (G), doped-graphene (doped-G) and control gold (Au) electrodes ( Fig. 2a ) have confirmed the improvement by doping. An order of magnitude decrease in electrode impedance with respect to an Au electrode was achieved at low frequencies. The reduction of impedance at low frequencies can have a big impact in suppressing electrical interference noise and electronic noise of the electrode itself. Effective surface areas of Au and graphene electrodes are expected to be very similar, as evaporated Au has a surface roughness less than 5 nm and graphene follows the surface roughness of underlying kapton substrate, which is less than 5 nm. 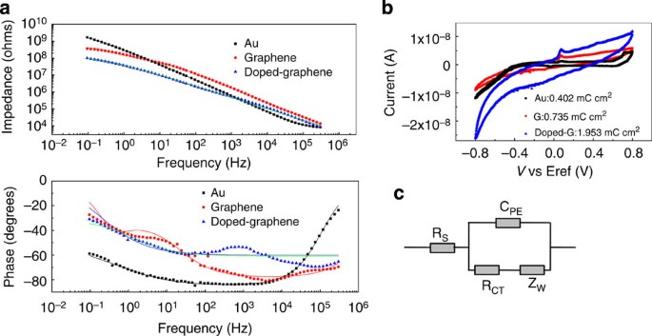Figure 2: Electrochemical characterization of graphene electrodes. (a) EIS results for 50 × 50 μm2Au, G and doped-graphene samples. Measurement results are shown with symbols and fitting results are shown with solid lines for impedance magnitude (top figure) and phase (bottom figure) plots. The impedance magnitude (top figure) significantly decreased with doping of graphene, more prominently for frequencies lower than 1 kHz. (b) Cyclic voltammogram showing enhanced charge storage capacity for doped-graphene electrode. Electrode size is 50 × 50 μm2. Legend shows calculated charge by integrating the area under the CV curve. (c) Schematic for the equivalent circuit model used to fit EIS measurement results.CPEis the constant phase element representing the double-layer capacitance;RCTis the charge transfer resistance;ZWis the Warburg element representing the diffusion of charges species to the interface andRSis the solution resistance. The models for circuit elements are provided inSupplementary Materials. Figure 2: Electrochemical characterization of graphene electrodes. ( a ) EIS results for 50 × 50 μm 2 Au, G and doped-graphene samples. Measurement results are shown with symbols and fitting results are shown with solid lines for impedance magnitude (top figure) and phase (bottom figure) plots. The impedance magnitude (top figure) significantly decreased with doping of graphene, more prominently for frequencies lower than 1 kHz. ( b ) Cyclic voltammogram showing enhanced charge storage capacity for doped-graphene electrode. Electrode size is 50 × 50 μm 2 . Legend shows calculated charge by integrating the area under the CV curve. ( c ) Schematic for the equivalent circuit model used to fit EIS measurement results. C PE is the constant phase element representing the double-layer capacitance; R CT is the charge transfer resistance; Z W is the Warburg element representing the diffusion of charges species to the interface and R S is the solution resistance. The models for circuit elements are provided in Supplementary Materials . Full size image The EIS curves for Au and G electrodes had different slopes, implying that the electrochemistry of the electrode interfaces can be different. The phase response of the Au electrode is capacitive (−90°) at low frequencies and becomes more resistive (0°) at higher frequencies. On the other hand, doped-G electrodes exhibit a much more complex phase response, where the phase angle remains constant around −50° for a wide range of frequencies. To better understand the electrochemical characteristics of graphene electrodes, EIS data were fit to an equivalent circuit model ( Fig. 2c ; Supplementary Table 1 ), where the interface is represented by a constant phase element in parallel with a resistor for faradaic charge transfer and a Warburg element for diffusion. Resistance of the phosphate-buffered saline (PBS) bath was modelled as a resistor in series with all other elements. The fitting results are plotted in Fig. 2a . The model provides a good fit for impedance results for all three types of electrodes. The phase response results show that the model works for Au and G electrodes at all frequencies. For the doped-G electrode, the model exhibit good fit for the impedance results, whereas some discrepancies between the model and the measurement are observed at higher frequencies for the complex phase response. The discrepancies in phase response observed only for doped-G samples suggest that charge transfer characteristics of doped graphene interface is more complex than Au and undoped graphene and shows some frequency dependency. The frequency dependency could be considered in the equivalent circuit model by adding another frequency-dependent capacitive component. However, for quantitative comparison, Table 1 lists the fitting results for the doped-G and Au electrodes according to the equivalent circuit model in Fig. 2d . The doped-G electrode has a much smaller charge transfer resistance and a more nonlinear constant phase element with a much larger constant, representing the capacitive nature of the interface. For neural recording electrodes, having a large interface capacitance helps reducing the electrode noise originating from the resistive charge transfer element [38] . Small charge transfer resistance accompanied with large capacitance for doped-G electrodes could help to suppress electronic noise, which was further investigated by in vivo neural recordings. Cyclic voltammetry (CV) measurements carried out on the same Au, G and doped-G electrodes also verified the improvement in the capacitive characteristics of doped-G electrode. Increased charge storage capacity for doped-G ( Fig. 2b ) could enhance the amount of transferred charge when graphene electrodes are used for neural stimulation applications [39] . Table 1 Fitting results for EIS measurements. Full size table In vivo neural recordings with graphene electrodes Lowering the electrode impedance by increasing the effective surface area [40] has been the most standard approach to improve the performance and scale down the sizes of extracellular microelectrodes. However, what really determines the electrode performance and its scalability to single-neuron dimensions is the ratio between the recorded neural signal and noise level, the SNR. Recent theoretical [41] , [42] and experimental [43] works have highlighted that impedance and microelectrode area are not as effective as previously thought in determining electrode performance. This is mainly because the thermal noise associated with the resistive component of electrode impedance is not the only noise source affecting neural recordings. Electronic noise in recording systems, biological noise and other noise sources associated with recording electrodes significantly degrade our ability to detect and sort neural signals. To better understand the SNR performance of graphene electrodes, we performed in vivo neural recording experiments on an adult rat animal model. In these experiments, an anaesthetized rat was placed with its head fixed in a stereotaxic apparatus. A craniotomy exposed a 4 × 8 mm 2 region of cortex in both hemispheres ( Fig. 3a ). To evoke epileptiform activity, crystals of bicuculline methiodide were applied directly to the recording site before electrode placement. As the aim of the experiment was to investigate the performance of graphene electrodes, single electrodes of various sizes were used instead of electrode arrays. Graphene electrode and Au control electrodes were placed in the left and right hemispheres to record simultaneously. 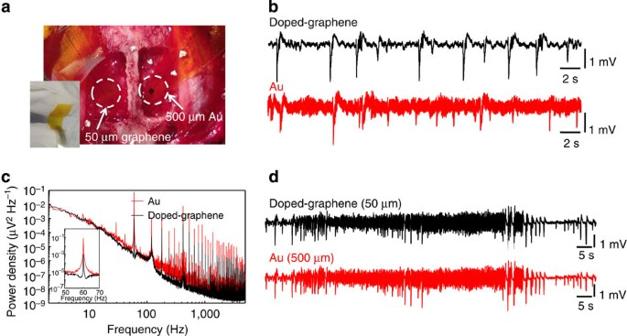Figure 3:In vivoneural recordings in rats. The data presented here are representative of three different acute experiments, each of them lasting 5–6 h. (a) The photograph of a 50 × 50 μm2single-graphene electrode placed on the cortical surface of the left hemisphere and a 500 × 500 μm2single-Au electrode placed on the cortical surface of the right hemisphere. The inset shows the flexibility of the electrodes. (b) Interictal-like spiking activity recorded by 50 × 50 μm2doped-graphene and Au electrodes. Both electrodes were placed on the same hemisphere and connected to the same amplifier channel in subsequent recordings. Data were filtered with a 0.1 Hz–3 kHz bandpass filter. Recordings with doped-graphene electrodes are five- to sixfold less noisy compared with the ones with same size Au electrode. (c) Power density spectra of the recordings shown inbcalculated over 20 s time window. Doped-graphene electrode recorded significantly lower 60 Hz noise and its harmonics. The inset shows almost two orders of magnitude decrease in 60 Hz electrical interference noise. (d) Seizure-like discharges recorded by 50 × 50 μm2doped-G and 500 × 500 μm2Au electrodes simultaneously according to the electrode placement shown ina. Similar SNR are observed for both recordings. Figure 3b shows the low-frequency interictal-like spiking activity recorded by 50 × 50 μm 2 doped-G and Au electrodes. Both electrodes were placed on the same hemisphere and connected to the same amplifier channel in subsequent recordings to ascertain that there are no electrode location or amplifier channel-related variations in the measurements. Recordings with doped-G electrodes were found to have five to six times less noise compared with the ones with the Au electrodes of the same size ( Fig. 3b ), although they have comparable impedance values at around 1 kHz. Root mean square (RMS) noise was measured as 30.99±1.15 μV and 165.64±17.87 μV for doped-G and Au electrodes, respectively. It is important to note that base noise levels for both electrodes could be further improved by better electrical shielding. The SNR for a given recording was calculated by dividing the signal amplitude by twice the RMS noise voltage (SNR=Signal Amplitude/(2 × RMS noise)). Mean SNR was determined to be 40.8 for doped-graphene electrode and 7.7 for Au electrodes in prolonged recordings. Undoped-graphene electrodes were also tested in in vivo recordings. They exhibited RMS noise in between doped-G and Au electrodes. Therefore, we focused on only doped-G electrodes for further analysis and simultaneous optical imaging and electrophysiology experiments. Figure 3: In vivo neural recordings in rats. The data presented here are representative of three different acute experiments, each of them lasting 5–6 h. ( a ) The photograph of a 50 × 50 μm 2 single-graphene electrode placed on the cortical surface of the left hemisphere and a 500 × 500 μm 2 single-Au electrode placed on the cortical surface of the right hemisphere. The inset shows the flexibility of the electrodes. ( b ) Interictal-like spiking activity recorded by 50 × 50 μm 2 doped-graphene and Au electrodes. Both electrodes were placed on the same hemisphere and connected to the same amplifier channel in subsequent recordings. Data were filtered with a 0.1 Hz–3 kHz bandpass filter. Recordings with doped-graphene electrodes are five- to sixfold less noisy compared with the ones with same size Au electrode. ( c ) Power density spectra of the recordings shown in b calculated over 20 s time window. Doped-graphene electrode recorded significantly lower 60 Hz noise and its harmonics. The inset shows almost two orders of magnitude decrease in 60 Hz electrical interference noise. ( d ) Seizure-like discharges recorded by 50 × 50 μm 2 doped-G and 500 × 500 μm 2 Au electrodes simultaneously according to the electrode placement shown in a . Similar SNR are observed for both recordings. Full size image Power density spectra of the recordings with doped-G and Au electrodes calculated over a 20-s time window are shown in Fig. 3c . The doped-G electrode achieved a significant reduction in 60 Hz electrical interference noise and its harmonics. The power of electrical interference noise was reduced approximately 100 times for the doped-G electrode. The suppression of the electrical interference noise for the doped-G electrode may result from the large interface capacitance and small charge transfer resistance found in EIS analysis. This noise suppression suggests a clear advantage for studying brain activity in the low local field potential range (LFP: 1–100 Hz), which includes information on slow synaptic potentials. Figure 3d shows a sample from experimentally induced ictal-like activity recorded by 50 × 50 μm 2 doped-G and 500 × 500 μm 2 Au electrodes simultaneously according to the electrode placement shown in Fig. 3a . Despite a ~25-fold difference in impedance at 1 kHz (Au(500 μm): 17.2 kΩ, Doped-G(50 μm): 541 kΩ), the two electrodes showed comparable RMS noise, confirming that the impedance and area are not the only factors determining the noise performance of the electrodes, as predicted by modelling and simulation studies [41] , [42] . In addition to bicuculline-induced epileptiform activity in rats, graphene electrodes were also tested in vivo to record cortical spontaneous electroencephalography (EEG) in feline model ( Supplementary Fig. 4 ) and to record somatosensory-evoked potential (SSEP) in anaesthetized rats with no drug application ( Supplementary Fig. 5 ). In the SSEP experiment, two types of working electrodes (standard tungsten electrode and transparent graphene electrode) were sequentially placed on the surface of the exposed barrel cortex to record the SSEP produced by the vibrissa stimulation. The evoked potential measured at the cortical surface by the tungsten and the graphene electrodes consisted of a fast negative waveform followed by a positive long-lasting slow wave [44] , consistently ( Supplementary Fig. 5 ). In vivo recordings with graphene electrodes demonstrate their ability to record physiological, stimulus-evoked or drug-induced neural activity with high SNR in the LFP band. Impedance and noise characteristics of graphene electrodes can be further improved by employing alternative doping approaches, micropatterning for increasing the density of active sites or surface functionalization of graphene [45] . Simultaneous calcium imaging and electrical recording In order to investigate the feasibility of imaging through transparent doped-graphene electrodes, we performed calcium imaging in hippocampal tissue slices by both confocal and two-photon microscopy. Calcium imaging is intentionally chosen as it provides single cell-level spatial resolution, complementary to temporal resolution of electrophysiological recordings. However, transparent graphene electrode technology can also be integrated with voltage-sensitive dye imaging, to compare the field recordings from large populations of neurons. We measured the transmission spectrum of graphene electrodes fabricated on a polyimide substrate and found that the graphene/polyimide is transparent above the wavelength of 450 nm ( Fig. 4a ). The transmission increases with decreasing substrate thickness and was limited mainly by the polyimide substrate. Hence, it can be further enhanced by using thinner or more transparent substrates such as polyethylene terephthalate and polyethylene naphthalate. Calcium indicator dyes such as Oregon Green BAPTA-1 AM (OGB-1) can be used to detect the increase in fluorescence intensity in neuronal cell bodies occurring as a result of calcium influx accompanying action potential firing [5] , [6] . For confocal microscopy, OGB-1 is excited at 488 nm (shown in dotted blue line in Fig. 4a ) and emits fluorescence between 500 and 600 nm with a peak around 520 nm (shown in green shading in Fig. 4a ). For two-photon microscopy, a 840-nm femtosecond laser pulse is used (shown in dotted red line in Fig. 4a ) to excite OGB-1. We built special imaging chambers to submerge and constantly perfuse hippocampal slices and the graphene electrodes in artificial cerebrospinal fluid (ACSF) for the confocal ( Fig. 4b and Supplementary Fig. 6 ) and two-photon microscopy ( Fig.4c ). Hippocampal slices from early postnatal rats (postnatal day 2–5) were stained with OGB-1, placed on top of a 50 × 50 μm 2 graphene electrode in the chamber, and imaged with an inverted confocal microscope. Neural activity recorded by the graphene electrode shows no light-induced artefacts due to excitation light ( Supplementary Fig. 7 ). 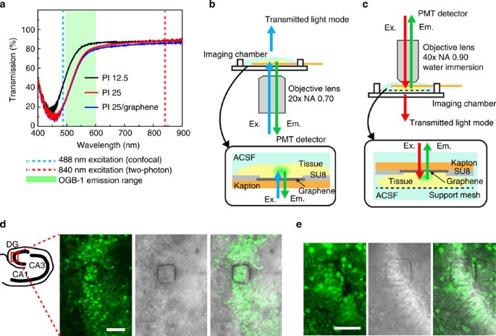Figure 4: Calcium imaging with confocal and two-photon microscopy setups. (a) Optical transmission spectrum of 12.5 and 25 μm bare Kapton films and 25 μm Kapton film coated with graphene. The fluorescence emission range of the calcium indicator dye, Oregon Green Bapta-1 (OGB-1) is shown in green shadow. The excitation wavelength (488 nm) used in the confocal microscopy is delineated by the dotted blue line. The excitation wavelength used in two-photon microscopy (840 nm) is delineated by the dotted red line. (b) Schematic illustration of the confocal microscopy setup with a custom imaging chamber for simultaneous imaging and recording. Insert: Hippocampus slice tissue was mounted on the graphene electrode and perfused with ACSF throughout the experiment. Note that excitation as well as emission light passes through the graphene electrode. (c) Schematic illustration of the two-photon microscopy setup with a custom imaging chamber. Two-photon microscopy operates with an upright microscope equipped with a high numerical aperture water immersion lens. Insert: In order to keep the slice tissue healthy, the custom chamber is equipped with a mesh support and the solution exchange occurs at the bottom of the tissue and the top of the electrode. (d) Left schematic shows different regions of the hippocampus. The dentate gyrus is imaged by the confocal microscope. Images show: Left: A steady-state fluorescence (F0) image of dentate gyrus in a OBG-1 AM-stained hippocampal slice obtained through the 50 × 50 μm2graphene electrode. The graphene electrode is seen as a square outline with dark edges. Middle: Simultaneously obtained transmittance image. Right: Merge of the steady-state fluorescence (right) and the transmittance images (left). Scale bar, 50 μm. (e) Dentate gyrus is imaged by the two-photon microscope. Images show: Left: A steady-state fluorescence (F0) image of dentate gyrus in a OBG-1 AM-stained hippocampal slice obtained through the 50 × 50 μm2graphene electrode. The graphene electrode is seen as a square outline with dark edges. Middle: Simultaneously obtained transmittance image. Right: Merge of the steady-state fluorescence (right) and the transmittance images (left). Scale bar, 50 μm. Figure 4d shows a steady-state fluorescence image of the dentate gyrus (DG) region captured through the graphene electrode. The exposed graphene electrode region, defined by the 50 × 50 μm 2 opening in the encapsulation layer, is seen as a square outline with dark edges ( Fig. 4d ). The excitation light at 488 nm as well as fluorescence emission (max at ~520 nm) penetrated through the 50 × 50 μm 2 transparent graphene electrode. Similarly, OGB-1-stained slices from early postnatal rats were placed in the chamber equipped with a support mesh and the graphene electrode was mounted on top of the slice for two-photon imaging on an upright microscope. Figure 4e shows a steady-state fluorescence image of the DG region imaged through the 50 × 50 μm 2 graphene electrode as visualized by two-photon microscopy. Approximately ten neuronal cell bodies overlapping with the electrode are clearly visible through the transparent graphene electrode. Figure 4: Calcium imaging with confocal and two-photon microscopy setups. ( a ) Optical transmission spectrum of 12.5 and 25 μm bare Kapton films and 25 μm Kapton film coated with graphene. The fluorescence emission range of the calcium indicator dye, Oregon Green Bapta-1 (OGB-1) is shown in green shadow. The excitation wavelength (488 nm) used in the confocal microscopy is delineated by the dotted blue line. The excitation wavelength used in two-photon microscopy (840 nm) is delineated by the dotted red line. ( b ) Schematic illustration of the confocal microscopy setup with a custom imaging chamber for simultaneous imaging and recording. Insert: Hippocampus slice tissue was mounted on the graphene electrode and perfused with ACSF throughout the experiment. Note that excitation as well as emission light passes through the graphene electrode. ( c ) Schematic illustration of the two-photon microscopy setup with a custom imaging chamber. Two-photon microscopy operates with an upright microscope equipped with a high numerical aperture water immersion lens. Insert: In order to keep the slice tissue healthy, the custom chamber is equipped with a mesh support and the solution exchange occurs at the bottom of the tissue and the top of the electrode. ( d ) Left schematic shows different regions of the hippocampus. The dentate gyrus is imaged by the confocal microscope. Images show: Left: A steady-state fluorescence (F0) image of dentate gyrus in a OBG-1 AM-stained hippocampal slice obtained through the 50 × 50 μm 2 graphene electrode. The graphene electrode is seen as a square outline with dark edges. Middle: Simultaneously obtained transmittance image. Right: Merge of the steady-state fluorescence (right) and the transmittance images (left). Scale bar, 50 μm. ( e ) Dentate gyrus is imaged by the two-photon microscope. Images show: Left: A steady-state fluorescence (F0) image of dentate gyrus in a OBG-1 AM-stained hippocampal slice obtained through the 50 × 50 μm 2 graphene electrode. The graphene electrode is seen as a square outline with dark edges. Middle: Simultaneously obtained transmittance image. Right: Merge of the steady-state fluorescence (right) and the transmittance images (left). Scale bar, 50 μm. Full size image Electrophysiological recordings were conducted in calcium indicator dye-loaded slices to explore the relationship between neuronal activity recordings from graphene electrodes and calcium transients. Potassium ion concentration was elevated to 6 mM (normally 3 mM), magnesium ion concentration was decreased to 0 mM (normally 2 mM), and 20 μM bicuculline-methiodide was added to ACSF to induce spiking activity. 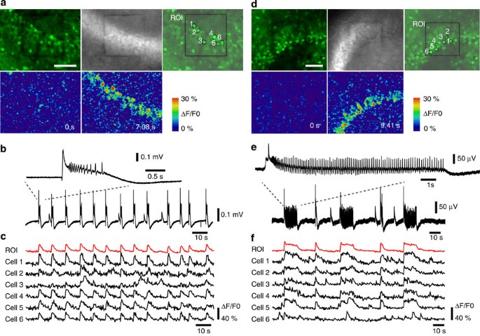Figure 5: Simultaneous multicellular calcium imaging and electrophysiology using transparent graphene electrodes. (a) Left: A steady-state fluorescence (F0) image of the dentate gyrus in a OBG-1 AM-stained hippocampal slice obtained by confocal microscopy. The excitation light at 488 nm as well as the fluorescence emission (max at ~520 nm) penetrated through the transparent electrode (graphene and polyimide substrate). Middle: Simultaneously obtained transmittance image. Right: Region of interest (ROI) for electrode area and randomly selected six cells within the electrode area are outlined. Calcium transients from these cells are shown inc. Bottom: Colour-coded images of normalized fluorescence change (ΔF/F0) at baseline (0 s) and during one of the peak responses (7.08 s). Scale bar, 50 μm. (b) Recording from the graphene electrode shows interictal-like activity, that is, short population bursts (shown in insert) that last less than a second, occurring every 5–12 s during the 2 min of recording. (c) The calcium transient (ΔF/F0) for the electrode area (labelled as ROI) shows an increase in calcium signal coinciding with the interictal-like event recorded inb. ΔF/F0 traces for individual cells show that most of the cells responded with the interictal-like event but with varied amplitude. Cell 2 did not respond to the third event. Cell 3 only responded to the forth event with a delayed peak. SeeSupplementary Movie 1. (d) Left: A steady-state fluorescence (F0) image of a different part of the dentate gyrus. Middle: Simultaneously obtained transmittance image. Right: ROI for electrode area and randomly selected six cells within the electrode area are outlined. Bottom: Colour-coded images of normalized fluorescence change (ΔF/F0) at baseline (0 s) and during one of the peak responses (9.41 s). Scale bar, 50 μm. (e) Recording from the graphene electrode shows ictal (seizure)-like activity, that is, prolonged population bursts (shown in insert) that lasted ~10 s, occurring three times during ~150 s of recording. (f) Calcium transients (ΔF/F0) for the electrode area (labelled ROI) increased to an elevated level (plateau) with respect to baseline during the ictal-like events. During the ictal-like event, cells 1, 2, 4 and 5 exhibited plateaus, whereas cells 3 and, 5 showed multiple peaks. Cell 6 did not participate in ictal-like activity. SeeSupplementary Movie 2. The data presented are representative of four differentin vitroexperiments performed on 12 rodent hippocampal slices. Figure 5a shows a steady-state fluorescence (F0) confocal microscopic image of the DG in a hippocampal slice from a P12 mouse stained with the calcium indicator OGB-1. The clear, in-focus edges of the exposed electrode region (a square outline with dark edges) indicate that the slice and the electrode are in close proximity. Electrophysiological recordings obtained with the graphene electrode ( Fig. 5b ) demonstrated interictal-like activity ( Supplementary Movie 1 ), that is, short population bursts (insert in Fig. 5b ) that lasted less than a second, occurring every 5–12 s during the 2 min of recording. Calcium transients (ΔF/F0) within the electrode area (labelled as region of interest (ROI), Fig. 5c ) captured by the confocal microscope show an increase in calcium signal coinciding with the interictal-like event recorded by the graphene electrode. The temporal resolution of the graphene electrode recordings enables detection of high-frequency population discharges, which cannot be resolved by the calcium fluorescence responses. In contrast, calcium imaging responses were able to capture complex network contributions of individual neurons, which were not evident in the electrical recordings. ΔF/F0 calcium imaging traces for individual cells ( Fig. 5c ) as well as a snapshot of ΔF/F0 movie (shown in Fig. 5a bottom right) show that most of the cells were activated during the interictal-like event with the amplitude reaching above 30%. Different from other cells, Cell 2 did not respond for the third event and the peak amplitude for each interictal event varied. Cell 3 was not active during most of the interictal-like events except for the fourth event. Figure 5d–f shows ictal (seizure)-like activity recorded in the same slice ( Supplementary Movie 2 ). During the ictal-like activity, the calcium transient for the electrode area (labelled as ROI) plateaued at an elevated level ( Fig. 5f ) with respect to baseline. Simultaneous graphene electrode recordings ( Fig. 5e ) resolved the ictal-like discharges onset, LFP and population bursts. Calcium transients from individual cells exhibited temporal differences in neuronal activity ( Fig. 5f ). In contrast to the other five cells, Cell 6 had an early response in the first ictal-like event, a late response in the second ictal-like event and late multiple responses during the last event. Figure 5: Simultaneous multicellular calcium imaging and electrophysiology using transparent graphene electrodes. ( a ) Left: A steady-state fluorescence (F0) image of the dentate gyrus in a OBG-1 AM-stained hippocampal slice obtained by confocal microscopy. The excitation light at 488 nm as well as the fluorescence emission (max at ~520 nm) penetrated through the transparent electrode (graphene and polyimide substrate). Middle: Simultaneously obtained transmittance image. Right: Region of interest (ROI) for electrode area and randomly selected six cells within the electrode area are outlined. Calcium transients from these cells are shown in c . Bottom: Colour-coded images of normalized fluorescence change (ΔF/F0) at baseline (0 s) and during one of the peak responses (7.08 s). Scale bar, 50 μm. ( b ) Recording from the graphene electrode shows interictal-like activity, that is, short population bursts (shown in insert) that last less than a second, occurring every 5–12 s during the 2 min of recording. ( c ) The calcium transient (ΔF/F0) for the electrode area (labelled as ROI) shows an increase in calcium signal coinciding with the interictal-like event recorded in b . ΔF/F0 traces for individual cells show that most of the cells responded with the interictal-like event but with varied amplitude. Cell 2 did not respond to the third event. Cell 3 only responded to the forth event with a delayed peak. See Supplementary Movie 1 . ( d ) Left: A steady-state fluorescence (F0) image of a different part of the dentate gyrus. Middle: Simultaneously obtained transmittance image. Right: ROI for electrode area and randomly selected six cells within the electrode area are outlined. Bottom: Colour-coded images of normalized fluorescence change (ΔF/F0) at baseline (0 s) and during one of the peak responses (9.41 s). Scale bar, 50 μm. ( e ) Recording from the graphene electrode shows ictal (seizure)-like activity, that is, prolonged population bursts (shown in insert) that lasted ~10 s, occurring three times during ~150 s of recording. ( f ) Calcium transients (ΔF/F0) for the electrode area (labelled ROI) increased to an elevated level (plateau) with respect to baseline during the ictal-like events. During the ictal-like event, cells 1, 2, 4 and 5 exhibited plateaus, whereas cells 3 and, 5 showed multiple peaks. Cell 6 did not participate in ictal-like activity. See Supplementary Movie 2 . The data presented are representative of four different in vitro experiments performed on 12 rodent hippocampal slices. Full size image In another example, the graphene electrode was able to measure very fast population spikes with durations less than 5 ms, as well as slow LFPs, which may corresponds to subthreshold synaptic activity. Those LFPs were not detectable by multicellular calcium imaging ( Supplementary Fig. 8 ). For some of the recordings, a standard patch pipette electrode was placed close to the edge of the graphene electrode to record field potentials. Neural activity recorded simultaneously by the graphene electrode and the patch electrode was found to be consistent ( Supplementary Fig. 9 ). Our experiments with hippocampal slices demonstrate that high-frequency activity, which cannot be observed by slow calcium transients in calcium imaging, can be detected in simultaneous graphene electrode recordings. Corrosion protection by graphene for electrode longevity In addition to low noise and transparency, graphene brings several other advantages, such as robustness, long-term stability and corrosion protection, to implantable microelectrode technologies. Corrosion of electrodes and impedance change over time have been two of the main issues degrading the long-term stability of neural microelectrode recordings. It has been recently demonstrated that graphene can act as a protective coating, which significantly reduces corrosion of underlying metals [31] , [32] by blocking the diffusion of molecules and corrosive electrochemical reactions at the metal interface in aqueous environments. To investigate the corrosion-protective characteristics of graphene, we carried out CV measurements on bare Au and G/Au bilayer electrodes, fabricated along with transparent graphene electrodes. The voltammogram for the bare Au electrode exhibits standard Au oxidation and reduction peaks ( Fig. 6a ), whereas the graphene-coated Au electrode does not show any faradaic reaction peaks. This confirms that graphene acts as a protective layer covering the Au electrode surface and inhibits electrochemical reactions. Because Au, as a noble metal, may not be the best material choice to study the corrosion protection characteristics of graphene, CV tests under the same conditions were repeated with Ag and G/Ag electrodes. Ag is a very corrosive electrode metal, which easily degrades through sulfidation and oxidation even when exposed to air. Because of its toxicity and instability, bare Ag cannot be used in neural implants. However, when coated with graphene, the electrochemical reactions at the Ag surface are eliminated. CV and potentiodynamic polarization tests show that graphene coating significantly reduced the Ag corrosion in PBS ( Supplementary Fig. 10 ). To examine the stability of graphene on metal surfaces, Raman spectroscopy was performed on G/Au samples dipped in PBS over an extended period of time ( Fig. 6b ). Clear graphene peaks after 11 days, 1 month and 6 months in saline show that graphene is stable on the electrode surface and the quality of graphene does not degrade over time in aqueous PBS solution. These findings suggest that graphene can be used as a corrosion-protective layer for metal microelectrodes to enhance long-term stability and robustness. 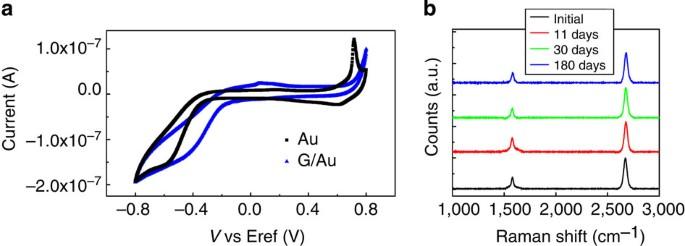Figure 6: Corrosion protection and inhibition of electrochemical reactions by graphene. (a) Cyclic voltammogram for Au and graphene-coated Au (G/Au) electrodes. G/Au sample does not exhibit any faradaic reaction peaks, showing that graphene acts as a protective layer covering Au surface. The electrode size is 500 × 500 μm2. (b) Raman spectroscopy measured on the same G/Au samples dipped it in PBS. Measurements were taken before dipping in PBS, after 11 days, after 30 days and after 6 months in PBS. Figure 6: Corrosion protection and inhibition of electrochemical reactions by graphene. ( a ) Cyclic voltammogram for Au and graphene-coated Au (G/Au) electrodes. G/Au sample does not exhibit any faradaic reaction peaks, showing that graphene acts as a protective layer covering Au surface. The electrode size is 500 × 500 μm 2 . ( b ) Raman spectroscopy measured on the same G/Au samples dipped it in PBS. Measurements were taken before dipping in PBS, after 11 days, after 30 days and after 6 months in PBS. Full size image Our results demonstrate that graphene electrodes enable simultaneous electrophysiological recording and optical imaging, combining the temporal and spatial resolution advantages of both techniques without perturbing either sensing mode. Electrical recordings with the graphene electrode successfully detected interictal and ictal activity, population discharges and fast population spikes with durations less than 5 ms, which cannot be resolved by multicellular calcium imaging. Capturing individual action potentials lasting 0.5–2 ms requires a temporal resolution of at least 0.25 ms. The temporal resolution of the graphene electrode recordings is only limited by the sampling frequency of the data acquisition setup, which is well beyond the requirements to detect action potentials. Spatial resolution can be further increased by scaling electrode dimensions to single-cell size through engineering the charge transfer characteristics and noise of graphene electrodes. The 5- to 6-fold improvement in SNR and 100-fold reduction in electrical interference noise demonstrated with 50 μm electrodes have already shown graphene’s potential to achieve that goal. In confocal microscopy studies, in order to compensate for the lower transmittance of the polyimide substrate at 488 nm, laser power was adjusted to about four times what is normally used for imaging bright fluorescence samples. For two-photon microscopy, this was not necessary, as the electrodes have high light transmittance at 840 nm. One of the advantages of using two-photon microscopy is the less toxic nature of near-infrared light compared with single photon light irradiation utilized in confocal microscopy. This effect is even more obvious when a ultraviolet-excitable dye is used. Selecting a substrate that has higher transmittance above 400 nm would be beneficial when using ultraviolet-excitable dyes as their emission usually ranges from 400 to 500 nm or above. Another advantage of two-photon microscopy is its capability to image deeper in the tissue, thus it is often used in in vivo imaging of mouse brains [2] , [4] , [5] . Combining in vivo two-photon imaging and cortical surface recording using flexible, transparent graphene electrode arrays present a viable approach to studying LFPs from the cortical surface simultaneously with neural activity from deeper layers. In recent work by Andermann et al . [46] , it was demonstrated that the entire cortical column was imaged in vivo in awake animals using two-photon microscopy with a prism implanted in the brain. Incorporation of various optical components and the graphene electrodes might be useful to probe deeper layers and larger areas in the brain tissue. Moreover, transparent graphene electrode arrays could be utilized for functional dynamic mapping of large cortical ensemble activity, such as in the visual cortex, by sequentially implementing two-photon imaging over a large area transparent array while simultaneously recording LFPs from the entire cortical surface. Such experiments would enable investigators to construct a comprehensive map of the visual cortex, multiscale. These experiments could relate how response dynamics in small networks control large-scale response propagation during visual stimulation with different statistical properties. Another interesting approach to linking cellular population activity to LFP network responses could be measuring high-frequency oscillations in epileptic networks while simultaneously investigating their origins with high-resolution two-photon microscopy. The techniques developed for single electrodes in this work can easily be extended to dense arrays in order to study larger areas. A combined sensing and imaging approach capable of simultaneously resolving both synaptic potentials and action potential firing with high spatial and temporal resolution in large populations of neurons could reveal circuit level behaviour and correlation between the activities in different parts of brain. Transparent graphene electrodes are also attractive for use with optogenetics, enabling simultaneous optical stimulation [47] of neural tissue. Optical stimulation in combination with multichannel electrophysiology has been a useful tool in assessing network dynamics [48] . However, light stimulation can cause considerable artefacts [49] in the recordings due to photoelectric effect in the metal microelectrodes, impeding effective recording of LFPs [50] , [51] . Use of graphene microelectrodes appears to completely eliminate this problem, offering artefact-free electrophysiology in combination with optical stimulation. Integrating simultaneous optogenetic stimulation, electrophysiological recording and optical imaging could potentially lead to paradigm shifts in understanding the connectivity and function of neural circuits. Moreover, because of the nonmagnetic nature of graphene, it can be easily integrated with functional magnetic resonance imaging and other imaging modalities. Beyond transparency and low noise, using graphene as a protective layer may allow us to leverage superior electrical characteristics of materials that are normally precluded from being used in implantable devices because of poor biocompatibility. These characteristics also might reduce the cost of implantable devices and prolong battery life in implantable devices, by allowing the use of more efficient conductors, that are immunoreactive when exposed, but safe when completely sealed by graphene. In summary, the flexible, transparent, low noise and resilient coating characteristics of the electrode technology presented in this paper could be a powerful tool in neuroscience linking low-level neuronal circuits to high-level brain function. The capability to record brain activity from a large number of neurons and interacting neural circuits, while simultaneously resolving individual cells and their connections through optical imaging, may greatly illuminate our understanding of how brain circuits process information. Graphene electrode fabrication Commercial polyimide films (Kapton, DuPont) with a thickness of 25 μm were attached to a temporary 4 inch Si carrier wafer coated with polydimethylsiloxane (PDMS), after cleaning it with acetone and isopropyl alcohol. In order to form metal electrodes and contact pads, Cr/Au (10 nm/100 nm) was deposited with thermal and electron-beam evaporation, respectively, on the kapton substrate previously patterned with photolithography. Following liftoff of the metal, chemical vapour deposition-grown graphene on Cu substrate was transferred onto the desired areas of the polyimide substrate in contact with the patterned Au pads using poly(methyl methacrylate) (PMMA)/PDMS stamping method ( Supplementary Fig. 1 ). The transferred graphene was patterned using photolithography and oxygen plasma etching. Finally, 7 μm SU-8 was deposited and patterned for encapsulation, covering all except the electrode areas. Nitric acid (70%) was used for chemical doping of certain graphene electrodes. As control samples, bare Au electrodes were fabricated in the same batch along with the G and G/Au bilayer electrodes using the same exact process except graphene transfer step. Anisotropic conductive film was bonded to the fabricated electrode contact pads to provide electrical connection to data acquisition system through a custom built interface board ( Supplementary Fig. 2 ). Electrochemical characterization EIS, CV and potentiodynamic polarization measurements were made using Gamry Reference 600 potentiostat/galvanostat/ZRA (Gamry Instruments). EIS measurements were made in standard three-electrode configuration and CV was made in two electrode configuration in 0.01 M PBS solution. Impedance measurements were taken between 0.01 Hz and 300 kHz using 10 mV RMS AC voltage. For CV tests, the potential on the working electrode was swept three times between −0.8 V and 0.8 V versus Ag/AgCl electrode in PBS solution at a scan rate of 200 mV s −1 , starting at the open circuit potential. The total charge transfer capability was calculated by taking time integral over the whole CV curve. To investigate the electrical characteristics of the electrode/electrolyte interface, we used the equivalent circuit model given in Fig. 2d , where R S is the solution resistance, C PE is a constant phase element representing the double-layer capacitor, R CT is faradaic charge transfer resistance and Z W is a Warburg element for diffusion. Equations for the equivalent circuit elements are listed in Supplementary Table I . Measured EIS results were fitted to equivalent circuit model to calculate the fit parameters for Au and doped_G electrodes. Porous bounded Warburg element was used to model the diffusion for Au electrode, whereas bounded Warburg element was used for doped_G electrode because it provided a better fit. Raman spectroscopy Raman spectra of the graphene-coated electrodes were taken using an NTEGRA Spectra (NT-MDT Co) system using a 532-nm laser excitation source. Optical transmission Transmission measurements of the Kapton films were taken using a Nikon TE-2000U (Nikon Corp.) inverted microscope with a white light source. Light transmitted through the samples was collected and coupled into a Shamrock SR-303i-B with a Newton EMCCD camera (Andor Technology plc.). In vivo neural recordings In vivo data presented in the paper ( Fig. 3 ) is representative of three different acute experiments, each of them lasting 5–6 h. The following procedures were approved by the Institutional Care and Use Committee of the University of Pennsylvania. In vivo experiments involved an anaesthetized rat with its head fixed in a stereotaxic apparatus. Wild-type, adult male and female rats were used in the experiments. The animal was anaesthetized with ketamine/xylazine throughout the craniotomy and neural recordings. A craniotomy exposed a 4 × 8 mm 2 region of cortex in both hemispheres. All recordings were taken in reference to a distant stainless steel bone screw inserted through the skull during the surgery. Neural data were acquired by a FHC multi-channel neural amplifier (FHC Inc. ) and an acquisition system (16 bit Axon Instruments Digidata 1322 A, Axon Instruments). Recordings were high pass filtered at 0.1 Hz. Neural recording data were analysed offline using Clampfit software (Axon Instruments). Slice preparation and staining Brains slices were prepared as described previously [52] . Briefly, the brains of male and female rats or mice (postnatal day 2-15 (P2-15)) were removed, glued to an agar block and sectioned (350 mm) in ice-cold ACSF containing the following (in mM): 130 sucrose, 3 KCl, 1.25 NaHPO 4 , 1 MgCl 2 , 2 CaCl 2 , 26 NaHCO 3 and 10 glucose. 10 μl of 10% pluonic acid (Lifetechnologies) in dimethylsulphoxide was added to 50 μg of Oregon Green BAPTA-1 AM (Lifetechnologies) and dissolved in 4 ml of ACSF (containing the following (in mM): 130 NaCl, 3 KCl, 1.25 NaH 2 PO 4 , 1 MgCl 2 , 2 CaCl 2 , 26 NaHCO 3 and 10 glucose) and 4 μl of 5% Cremophor EL (Sigma) in dimethylsulphoxide. The slices were submerged in a chamber equipped with a stirring bar in a water bath with 95% oxygen/5% carbon dioxide, and maintained at 37 °C for 30 min. Slices were washed and incubated in oxygenated ACSF at room temperature for at least 30 min before imaging. Live slice imaging A slice and an electrode were mounted in custom imaging chambers (modified from commercially available slice recording chambers (Warner Instruments)) and continuously perfused with ACSF or a modified ACSF containing the following (in mM): 130 NaCl, 6 KCl, 1.25 NaH 2 PO 4 , 26 NaHCO 3 , 0 MgCl 2 , 2 CaCl 2 , 10 glucose w/wo 20 μM of 1(S),9(R)-(-)-bicuculline methiodide (Sigma) and continuously bubbled with 95% O 2 /5% CO 2 . Slices were imaged on an Olympus Fluoview 1000 Laser Scanning Confocal Microscope equipped with a × 20 UPlanApo objective lens (numerical aperture=0.70). We focused on a region of area CA3 or DG. A time-series movie of fluorescence images was captured, generated by excitation light at 488 nm, eliciting emission between 500 and 600 nm. Transmittance images were captured simultaneously with the fluorescence images. The confocal microscope provided acquisition speed of 2–5 Hz with about 250 × 200 pixel imaged areas. For two-photon microscopy, images were acquired using a Prairie Technologies Ultima multiphoton system attached to an Olympus BX-61 upright microscope. Excitation light was provided by a diode-pumped broadband mode-locked titanium:sapphire femtosecond laser (SpectraPhysics, MaiTai HP 690–1040, <100 fs, 80 MHz). The laser beam was focused on the specimen by a × 40 water-immersion objective (numerical aperture=0.90, LUMPlanFL/IR, Olympus). An excitation wavelength of 840 nm was used. Emitted fluorescence was collected with the same objective lens, reflected by a dichroic filter (660LP) passing through in infrared cut filter (650SP; Chroma Technology); and detected with a photomultiplier tube (Hamamatsu). Neural recordings with the graphene electrodes were acquired by a CyberAmp 380 neural amplifier and acquisition system (Axon Instruments) with a Ag/AgCl pellet used as a bath electrode. A 60 Hz noise eliminator (HumBug, AutoMate Scientific) was used to reduce electrical line noise interference. Neural recording data were analysed offline using Clampfit software (Axon Instruments). Image analysis All images were processed using FIJI or NIH ImageJ software. For calcium transient traces, ROIs corresponding to somata were selected manually and the average intensity of ROIs was calculated. Custom written Matlab (Mathworks) codes were used to calculate background subtracted normalized fluorescence change (ΔF/F 0 ). 3 × 3 median filter was used when generating colour-coded ΔF/F 0 movies. How to cite this article: Kuzum, D. et al . Transparent and flexible low noise graphene electrodes for simultaneous electrophysiology and neuroimaging. Nat. Commun. 5:5259 doi: 10.1038/ncomms6259 (2014).